Excitation-dependent visible fluorescence in decameric nanoparticles with monoacylglycerol cluster chromophores Organic fluorescent nanoparticles, excitation-dependent photoluminescence, hydrogen-bonded clusters and lysobisphosphatidic acid are four interesting individual topics in materials and biological sciences. They have attracted much attention not only because of their unique properties and important applications, but also because the nature of their intriguing phenomena remained unclear. Here we report a new type of organic fluorescent nanoparticles with intense blue and excitation-dependent visible fluorescence in the range of 410–620 nm. The nanoparticles are composed of ten bis(monoacylglycerol)bisphenol-A molecules and the self-assembly occurs only in elevated concentrations of 2-monoacylglycerol via radical-catalysed 3,2-acyl migration from 3-monoacylglycerol in neat conditions. The excitation-dependent fluorescence behaviour is caused by chromophores composed of hydrogen-bonded monoacylglycerol clusters, which are linked by an extensive hydrogen-bonding network between the ester carbonyl groups and the protons of the alcohols with collective proton motion and HO···C=O (n→π*) interactions. Over the past few years, metal-free or organic fluorescent nanoparticles [1] have received considerable attention because of their potential applications in biology and the material sciences due to some of their advantages, including a low biological toxicity and being environmentally friendly. In addition, excitation-dependent photoluminescence (excitation-dependent fluorescent, EDF) [2] , which is an intriguing photoluminescence phenomenon exhibited by carbon-based nanoparticles, has received considerable interest. Several pioneering examples, including graphene [2] , [3] , [4] , graphite [5] , [6] , diamonds [7] , [8] , carbon nanotubes [9] , combustion candle soot [10] and pyromellitic diimide nanowire [11] , have recently been reported in the literature. Although a number of mechanisms have been suggested, the origin of the excitation-dependent photoluminescence remains unclear. The mechanisms for the formation and stabilization of spherical organelles via the self-assembly of phospholipids is one of the most important subjects in molecular cell biology. Lysobisphosphatidic acid (LBPA, Fig. 1a ), which is also called bis(monoacylglycerol)phosphate, is an unconventional phospholipid that possesses two monoacylglycerol moieties, is found in elevated concentrations in the late endosomes and lysosomes and is believed to have a significant role in the formation of the intraendosomal vesicular bodies [12] , [13] . It is not clear how the active form of LBPA adopts the less thermodynamically stable 2,2′-positional rather than the 3,3′- positional isomer [14] , or what the mechanisms are for the formation and transformation of the 2,2′-LBPA. 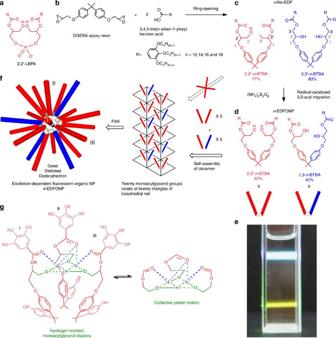Figure 1: Self-assembly of excitation-dependent visible fluorescent bis(monoacylglycerol)bisphenol-A decameric nanoparticles with monoacylglycerol cluster chromophores. (a) Structure of 2,2′-lysobisphosphatidic acid (2,2′-LBPA). (b) Reactants. (c) Initial products ofn-No-EDF (due to no EDF behaviour): two kinetically controlled products, 2,2′-n-BTBA and 3,3′-n-BTBA in a ratio of 17:83, are obtainedviaa ring-opening reaction in the first stage. (d)n-EDFONP: the concentration of 2-monoacylglycerol moiety of 2,2′-n-BTBA and 2,3-n-BTBA is increased from 17 to 60% after the radical-catalysed 3,2-acyl migration reaction in the second stage. (e) Intense blue (up) and yellow (down) fluorescences excited by a 405 nm violet and a 532 nm green light laser diodes, respectively. (f) Formation of Great Stellated Dodecahedral decamers by the self-assembly of five 2,2′-n-BTBA and five 2,3-n-BTBA. (g) Formation of the cyclic hydrogen-bonded monoacylglycerol clusters with collective proton motion (green line and dash) within three adjacent monoacylglycerol groups (I, II and III). Figure 1: Self-assembly of excitation-dependent visible fluorescent bis(monoacylglycerol)bisphenol-A decameric nanoparticles with monoacylglycerol cluster chromophores. ( a ) Structure of 2,2′-lysobisphosphatidic acid (2,2′-LBPA). ( b ) Reactants. ( c ) Initial products of n -No-EDF (due to no EDF behaviour): two kinetically controlled products, 2,2′- n -BTBA and 3,3′- n -BTBA in a ratio of 17:83, are obtained via a ring-opening reaction in the first stage. ( d ) n -EDFONP: the concentration of 2-monoacylglycerol moiety of 2,2′- n -BTBA and 2,3- n -BTBA is increased from 17 to 60% after the radical-catalysed 3,2-acyl migration reaction in the second stage. ( e ) Intense blue (up) and yellow (down) fluorescences excited by a 405 nm violet and a 532 nm green light laser diodes, respectively. ( f ) Formation of Great Stellated Dodecahedral decamers by the self-assembly of five 2,2′- n -BTBA and five 2,3- n -BTBA. ( g ) Formation of the cyclic hydrogen-bonded monoacylglycerol clusters with collective proton motion (green line and dash) within three adjacent monoacylglycerol groups (I, II and III). Full size image Here we report a series of bis(monoacylglycerol) decameric nanoparticles with intense blue and excitation-dependent visible fluorescence. The self-assembly of nanoparticles only occurs when the concentration of 2-monoacylglycerol is increased from ~17% to ~61%, which is analogous to the formation of intraendosomal vesicles in the late endosomes. Therefore, the bis(monoacylglycerol) bisphenol-A molecules resemble LBPA not only because both are wedge-shaped and possess two monoacylglycerol moieties, but most important, because both are ‘functional active’ when the amount of 2-monoacylglycerol increases from ‘functional inactive’ 3-monoacylglycerol form in the spherical aggregation through 3,2-acyl migration. The results from the experiments and theoretical calculations indicate that the radical-induced 3,2-acyl migration reactions may occur more readily for monoacylglycerol groups. These results also highlight important roles of 2-monoacylglycerol, hydrogen-bonded monoacylglycerol clusters, collective proton motion and HO···C=O (n→π*) interactions in the stabilization of nanoparticles and in the mechanism of EDF phenomenon. The concept of monoacylglycerol cluster-induced excitation-dependent visible fluorescence can be generalized to polymer systems. We expect that the results we report here can provide a new direction for designing and fabrication of low-toxicity visible fluorescent nanomaterials without an extended conjugated system via ‘green’ synthesis. We also hope that these results may facilitate our understanding of the role of monoacylglycerol-containing lipids in biology, such as the formation and mechanism of 2,2′-LBPA in late endosomes. Characterization and formation mechanism The initial products, which are abbreviated as n -No-EDF ( Fig. 1c ) because no EDF behaviour is observed, are obtained via a ring-opening reaction by treating the diglycidyl ether of bisphenol-A epoxy resin with the 3,4,5-tris( n -alkan-1-yloxy)benzoic acids ( Fig. 1b ). Both the 2,2′- n -BTBA and the 3,3′- n -BTBA are identified through 1 H, 13 C, heteronuclear single quantum correlation (HSQC) and heteronuclear multiple bond correlation (HMBC) NMR experiments ( Supplementary Figs S1–S3 ). The ratio of 17 and 83% is typical for kinetically controlled reactions [15] because the 3-position contains less steric hindrance than the 2-position. A subsequent radical-catalysed 3,2-acyl migration reaction is conducted by treating the initial products, n -No-EDFs, with 0.13 equiv. ammonium persulfate ((NH 4 ) 2 S 2 O 8 ) as a catalyst under neat conditions at 150 °C for 38 h. The products resulting from the migration of the 3,2-acyl, which are abbreviated as n -EDFONP ( Fig. 1d ), are also identified through 1 H, 13 C, HSQC and HMBC NMR spectra, but their NMR spectra are significantly different from that of the n -No-EDFs. The 1 H signals of the 12 -EDFONP in CDCl 3 at 10 mM are composed of ~80% broad and 20% sharp signals ( Supplementary Figs S4–S11 ). The dominant broad NMR signals are assigned to 2,2′- 12 -BTBA (40%) and 2,3- 12 -BTBA (40%), and they have significant upfield or downfield shifts compared with that of the initial 12 -No-EDF. The remaining 20% sharp signals correspond to free 2,2′- 12 -BTBA (1%), 3,3′- 12 -BTBA (15%) and 2,3- 12 -diacylglycerol-bisphenol-glycerol isomer (4%, a phosphatidylglycerol-like compound). These broad signals are attributed to the extremely dense aggregated structures, in which the internal conformational mobility is reduced [16] . In contrast, all of the 1 H NMR signals corresponding to 2,2′- 12 -BTBA and 3,3′- 12 -BTBA in the 12 -No-EDF in CDCl 3 at 10 mM are normally sharp, which indicates no dense aggregated structure being formed in the low concentration of 2,2′- 12 -BTBA. In other words, the increased concentration of the 2-monoacylglycerol moieties in the 12 -EDFONP from ~17% to ~61% after the 3,2-acyl migration causes the formation of dense aggregated structures with a yield of 80%. To determine whether the acyl migration is caused by the sulphate radical or the basicity of the sulphate, one reaction was performed by replacing (NH 4 ) 2 S 2 O 8 with potassium carbonate (K 2 CO 3 ) under the same reaction conditions. The results indicated that only a small amount of 2,3-diacylglycerol-bisphenol-glycerol was obtained; however, no 2,2′-isomer was observed ( Supplementary Fig. S12 ). Therefore, the radical-catalysed 3,2-acyl migration was established. The results from theoretical calculations at the M06-2x (ref. 17 )/cc-pVDZ level indicate that the activation energy of the alkoxy radical-induced acyl migration mechanism is 1.8 kcal/mol less than the migration by the hydroxyl form ( Supplementary Fig. S13 ). Therefore, the 3,2-acyl migration is readily able to occur via the alkoxy radical pathway. Characterization and properties of EDF organic nanoparticles Investigations based on the combination of NMR, high-resolution transmission electron microscopy (HRTEM), dynamic light scattering (DLS) and photoluminescence spectra reveal that the densely aggregated structures of the acyl-migrated product are discrete self-assembled EDF organic nanoparticles ( n -EDFONPs). The HRTEM image of 18 -EDFONP with a diameter of ~7.6 nm is shown in Fig. 2a . The mean diameters of 12 -EDFONP to 18 -EDFONP in CH 2 Cl 2 measured using DLS are 4.8, 6.0, 8.6 and 9.5 nm ( Supplementary Fig. S14 ). All of the n -EDFONPs have a similar photoluminescence excitation and emission behaviour in CH 2 Cl 2 and CHCl 3 solvents. In the case of 12 -EDFONP in CHCl 3 at a concentration of 10 mM, the excitation spectrum exhibits a broad peak at 330 nm with a shoulder that extends to ~650 nm ( Fig. 2b ). The excitation of 12 -EDFONP from 360 to 600 nm results in an EDF from 415 to 660 nm, where the intensity remarkably decreases ( Fig. 2b ). The quantum yield is determined to be 8.3% with coumarin 1 as a reference and the fluorescence lifetime measurement of the excitations of 12 -No-EDF at 329 nm and 12 -EDFONP at 360 nm are determined to be 0.98 and 1.54 ns, respectively ( Supplementary Fig. S15 ). Figure 1e is a fluorescent photograph of 12 -EDFONP in a CH 2 Cl 2 solution, which was simultaneously excited at 405 and 532 nm and exhibits intense blue and yellow fluorescences in the same quartz cuvette. In contrast, the excitation spectrum of 12 -No-EDF at a concentration of 10 mM displays only one excitation peak at 329 nm and one corresponding relatively shaper ultraviolet fluorescence peak at 353 nm ( Fig. 2c ). However, when the concentrations of 12 -EDFONP and 12 -No-EDF are subsequently decreased from 10 to 0.01 mM by dilution, both exhibit similar excitation and emission spectra ( Fig. 2c ). Two excitation peaks at 235 and 274 nm and one emission peak at 355 mM (excited at 274 nm) were observed, which indicated that both 12 -EDFONP and 12 -No-EDF dissociated into individual 3,3′- 12 -BTBA and 2,2′- 12 -BTBA molecules without dense aggregation when diluted to a concentration of 0.01 mM. The emission behaviour of 12 -No-EDF in high and low concentrations is typical of J-aggregate emission [18] . However, when 12 -EDFONP is reconcentrated from 0.01 to 10 mM, the broad characteristic excitation and EDF reappears (spectrum in green in Fig. 2d ). This result clearly indicates that the EDF behaviour is induced by the dense aggregation in the self-assembled organic nanoparticles but not by the individual n -BTBA molecule itself. To determine the functional groups—including bisphenol, benzoate and monoacylglycerol—that are responsible for the EDF behaviour, two compounds were prepared by changing the benzoate and bisphenol-A groups to the heptadecyl carboxylate and n -butyl glycidyl ether groups, respectively ( Supplementary Figs S16 and S17 ). Both of the modified compounds also exhibited the EDF behaviour ( Fig. 2e ), which clearly indicates that the 2-monoacylglycerol group is responsible for the EDF behaviour. In addition, this result also indicates that the EDF behaviour is a common phenomenon for the 2-monoacylglycerol-dominated compounds. Note that the bis(monoacylglycerol) clusters serve as chromophores here without any extended conjugated system. 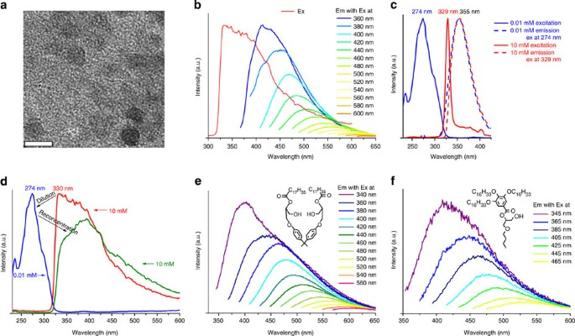Figure 2: Image and fluorescence spectra of EDFONPs. Spectroscopy performed in CHCl3. (a) HRTEM image of18-EDFONP with a scale bar of 10 nm. (b) Excitation and emission spectra of12-EDFONP at a concentration of 10 mM with a excitation-dependent visible fluorescence from 410 to 620 nm. (c) Excitation and emission spectra of12-No-EDF at concentrations of 0.01 and 10 mM. (d) Excitation spectra of12-EDFONP at an initial concentration of 10 mM (red line), then diluted to 0.01 mM (blue line) and reconcentrated back to 10 mM (green line). (e) Emission spectrum of17-EDFONP based on stearic acid at a concentration of 10 mM with a visible EDF phenomena. (f) Emission spectrum of16-EDFONP-BGE at a concentration of 10 mM with a visible EDF phenomena. Figure 2: Image and fluorescence spectra of EDFONPs. Spectroscopy performed in CHCl 3 . ( a ) HRTEM image of 18 -EDFONP with a scale bar of 10 nm. ( b ) Excitation and emission spectra of 12 -EDFONP at a concentration of 10 mM with a excitation-dependent visible fluorescence from 410 to 620 nm. ( c ) Excitation and emission spectra of 12 -No-EDF at concentrations of 0.01 and 10 mM. ( d ) Excitation spectra of 12 -EDFONP at an initial concentration of 10 mM (red line), then diluted to 0.01 mM (blue line) and reconcentrated back to 10 mM (green line). ( e ) Emission spectrum of 17 -EDFONP based on stearic acid at a concentration of 10 mM with a visible EDF phenomena. ( f ) Emission spectrum of 16 -EDFONP-BGE at a concentration of 10 mM with a visible EDF phenomena. Full size image Decamer and hydrogen-bonded monoacylglycerol cluster Further structural characterization using matrix-assisted laser desorption ionization time-of-flight mass spectrometry (MALDI-TOF-MS), NMR, Fourier transform infrared (FT-IR) experiments and theoretical calculations indicate the formation of decamers that contain a hydrogen-bonded monoacylglycerol clustered structure with collective proton motion. The MALDI-TOF-MS spectra of the n -EDFONPs reveal a group of signals that exhibit the pattern of an arithmetic series corresponding from a monomer to a decamer. For example, Fig. 3a shows the MALDI-TOF-MS spectrum of the 18 -EDFONP, which exhibits an ion peak at m/z =21,856 ([M 10 -6H 2 O+Na] + ) that corresponds to the decamer losing six water molecules. It is well known that dehydration is typical for hydroxyl-containing compounds in MALDI-TOF-MS experiments. In addition, a group of signals with an arithmetic series pattern corresponding to the decamer to tetramer losing water molecules. There are six ion peaks (A–F) to be observed between n -mers, which attributed to several fragment eliminations after acyl migration during the ionization process. The diffusion coefficient is measured using the NMR DOSY technique for solutions of 18 -EDFONP. The spectrum shows only one diffusion species that is characterized by the diffusion coefficient, D , of 0.95 × 10 −10 m 2 s −1 ( Supplementary Fig. S18 ) and the hydrodynamic radius of 3.9 nm is calculated from the Stokes–Einstein equation: r H = k B T /6π ηD , where k is the Boltzmann constant, T is the temperature, η is the viscosity of solution. The molecular weight of 18 -EDFONP is estimated to be ~24,000 from the Mark–Houwink–Sakaruda equation of D =2.45 (± 0.04) 10 −4 Mw −(0.55 ± 0.05) , which is determined by the phenolphthalein poly(ether sulphone) in chloroform solution. [19] By combining this result with the MALDI-TOF-MS spectrum, it was suggested that the formation of a decamer. Because the ratio of 2,2′- n -BTBA and 2,3- n -BTBA determined using 1 H NMR is ~1:1, the decamer should be composed of five 2,2′- n -BTBA and five 2,3- n -BTBA, fifteen 2-monoacylglycerol and five 3-monoacylglycerol moieties, specifically ( Fig. 1d ). These 20 monoacylglycerol moieties could construct a Great Stellated Dodecahedral ( Fig. 1f ), in which every three neighbouring monoacylglycerol groups form a triangular unit ( Fig. 1f , 2-monoacylglycerol I, II and III). The 1 H and 13 C NMR and liquid FT-IR spectra reveal the formation of dynamic hydrogen-bonded alcohol clusters with collective proton motion within each triangular unit ( Fig. 1g ). Remarkable differences in both the 13 C and 1 H chemical shifts are observed in the comparison of the 12 -EDFONP and 12 -No-EDF spectra. In the spectrum for the 12 -EDFONP, the 13 C signals of the hydroxyl-bearing carbon of 2,2′- 12 -BTBA and 2,3- 12 -BTBA undergo a downfield shift of approximately 7.0 and 7.5 p.p.m., respectively, relative to the signals of both BTBAs without dense aggregation in 12 -No-EDF ( Fig. 3b and Supplementary Fig. S7 ). The Δ δ 7.0 and 7.5 p.p.m. downfield shifts are typical for the hydroxyl-bearing carbons of polyvinyl alcohol and are characteristic of the formation of oligomeric alcohol clusters through continuous alcohol O-H···O-H hydrogen bonding [20] . The 1 H signals of the hydroxyl protons are no longer present in the 12 -EDFONP, and these signals are broadened and shifted downfield to 6.2–6.6 p.p.m. for the other three n -EDFONP ( n =14, 16 and 18; Supplementary Fig. S5 ) relative to sharp signals at 2.75 p.p.m. for the 12 -No-EDF ( Supplementary Fig. S1 ). 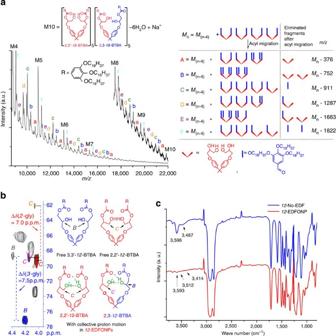Figure 3: Characterization of decamer and hydrogen-bonded monoacylglycerol cluster. (a) MALDI-TOF-MS of18-EDFONP shows an arithmetic series ion peaks corresponding to the decamer to tetramer with dehydration. Inset spectrum is amplification of the higher mass region. There are six ion peaks (A–F) to be observed betweenn-mers that attributed to several fragment eliminations after acyl migration during the ionization process. (b) Part of the1H–13C HSQC spectrum of12-EDFONP; the13C signals of the hydroxyl-bearing carbon atoms (H-C-OH···OH) of the 3- and 2-monoacylglycerol groups in the hydrogen-bonded monoacylglycerol cluster are significantly shifted downfield by approximately 7.5 and 7.0 p.p.m., respectively, compared with both in solution. (c) Liquid FT-IR spectra of12-No-EDF (blue line) and12-EDFONP (red line) at a concentration of 10 mM in CH2Cl2at room temperature. The dramatic decrease in the intensity of the two bands at 3,596 and 3,487 cm−1indicates the formation of cooperative hydrogen-bonded alcohol clustering with collective proton motion. Figure 3c shows the liquid FT-IR spectra of 12 -EDPONP and 12 -No-EDF in CH 2 Cl 2 . The primary difference between these two spectra is the O-H band region at 3,300–3,650 cm −1 . In the 12 -No-EDF spectrum, one terminal O-H band at 3,596 cm −1 and one hydroxyl dimer broadband at 3,487 cm −1 were observed [21] . However, in the 12 -EDPONP spectrum, only three very weak bands, including one terminal O-H band at 3,593 cm −1 , one hydroxyl dimer at 3,512 cm −1 and one cyclic hydroxyl trimer band at 3,414 cm −1 , were observed. The dramatic decrease in the intensity of the former two bands accounts for the formation of cooperative alcohol O-H···OH hydrogen-bonding networks with collective proton motions, which result in very weak OH stretching bands [22] . The results from theoretical calculations at the M06-2X/cc-pVDZ level for three acetyl 2-monoacylglycerolbenzene molecules as a static model reveal that the hydrogen-bonded cyclic alcohol trimer is 33.3 kcal mol −1 more stable than that of the three discrete acetyl 2-monoacylglycerolbenzene molecules, which is indicative of stabilization by cooperative alcohol hydrogen bonding ( Fig. 4a and Supplementary Fig. S19 ). Therefore, the cyclic 2-monoacylglycerol trimer can serve as a triangular-shaped building block with a large curvature leading to an n -EDPONP via spherical aggregation. In contrast, the result of theoretical calculations for the 3-monoacylglycerol trimer cluster using the same UM06-2x/cc-pVDZ method used for the 2-monoacylglycerol trimer cluster ( Supplementary Fig. S19d ) reveals that the three 3-monoacylglycerol molecules are nearly parallel and could not contribute to the curvature leading to the formation of the spherical aggregate. Because the primary difference between 2-monoacylglycerol and 3-monoacylglycerol is the hydroxyl group, it is either a primary R 2 CHCH 2 OH or secondary R 2 CHOH group. Considering the length between O and tertiary C atoms and flexibility, the former is not only longer (2.477 Å in Supplementary Fig. S19c ) than the latter (1.406 Å in Supplementary Fig. S19d ), but also more rotationally flexible. In addition, apparently the angles between the hydroxyl O atom, tertiary C atom and methyl C atom in the 2-monoacylglycerol and 3-monoacylglycerol trimers are 104 and 73° ( Supplementary Fig. S19c,d ), which clearly indicate that the 2-monoacylglycerol group is more suitable for the formation of a spherical aggregate than the 3-monoacylglycerol group. Figure 3: Characterization of decamer and hydrogen-bonded monoacylglycerol cluster. ( a ) MALDI-TOF-MS of 18 -EDFONP shows an arithmetic series ion peaks corresponding to the decamer to tetramer with dehydration. Inset spectrum is amplification of the higher mass region. There are six ion peaks (A–F) to be observed between n -mers that attributed to several fragment eliminations after acyl migration during the ionization process. ( b ) Part of the 1 H– 13 C HSQC spectrum of 12 -EDFONP; the 13 C signals of the hydroxyl-bearing carbon atoms (H- C -OH···OH) of the 3- and 2-monoacylglycerol groups in the hydrogen-bonded monoacylglycerol cluster are significantly shifted downfield by approximately 7.5 and 7.0 p.p.m., respectively, compared with both in solution. ( c ) Liquid FT-IR spectra of 12 -No-EDF (blue line) and 12 -EDFONP (red line) at a concentration of 10 mM in CH 2 Cl 2 at room temperature. The dramatic decrease in the intensity of the two bands at 3,596 and 3,487 cm −1 indicates the formation of cooperative hydrogen-bonded alcohol clustering with collective proton motion. 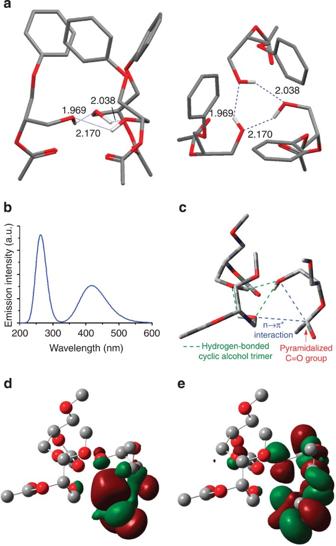Figure 4: TD-DFT calculation of trimeric monoacylglycerol cluster. (a) Optimized ground-state geometries of cyclic hydrogen-bonded acetyl 2-monoacylglycerolbenzene trimer at M06-2X/cc-pVDZ level viewed from side (left) and top (right) directions. The hydrogen atoms except that of hydroxyl groups are omitted for clarity. (b) Calculated emission spectrum. (c) Optimized excited state geometry at UM06-2x/6-31g(d) with TD-DFT method based on the optimized ground-state structure of the second excited state at UM06-2X/6-31g(d) level. One carbonyl group was pyramidalized due to two n→π* interactions with two adjacent alcohol O atoms (blue dash lines). (d) LUMO orbital and (e) HOMO orbital were dominated by carbonyl π* and non-bonding orbitals, respectively, as well as the adjacent OH non-bonding orbitals. The unit of bond length is angstrom. Full size image Figure 4: TD-DFT calculation of trimeric monoacylglycerol cluster. ( a ) Optimized ground-state geometries of cyclic hydrogen-bonded acetyl 2-monoacylglycerolbenzene trimer at M06-2X/cc-pVDZ level viewed from side (left) and top (right) directions. The hydrogen atoms except that of hydroxyl groups are omitted for clarity. ( b ) Calculated emission spectrum. ( c ) Optimized excited state geometry at UM06-2x/6-31g(d) with TD-DFT method based on the optimized ground-state structure of the second excited state at UM06-2X/6-31g(d) level. One carbonyl group was pyramidalized due to two n→π* interactions with two adjacent alcohol O atoms (blue dash lines). ( d ) LUMO orbital and ( e ) HOMO orbital were dominated by carbonyl π* and non-bonding orbitals, respectively, as well as the adjacent OH non-bonding orbitals. The unit of bond length is angstrom. Full size image TD-DFT calculation We suggest that the EDF phenomenon is caused by the combination of dynamically hydrogen-bonded alcohol clusters with collective proton motion and excited-state HO···C=O (n→π*) interactions, which can be regarded as a Bürgi–Dunitz trajectory [23] interaction (Nu···C=O interactions). The existence of O···C=O interactions have been confirmed by protein structures [24] , [25] , [26] and small molecules [27] , and they have a significant role in the stabilization of collagen [28] and the α-helix [29] . The fluorescence spectrum was calculated using the TD-DFT/UM06-2X/6-31g(d) method based on the optimized structure of the second excited state of the cyclic acetyl-2-monoacylglycerolmethane trimer at the UM06-2X/6-31g(d) level, and it is shown in Fig. 4b . The result from the calculation predicts two emission peaks at 263 and 418 nm. The latter is consistent with the experimental value. Note that the LUMO (S 1 ) is dominated by the π* orbital of the C=O group with a significant pyramidalization ( Fig. 4c ). In addition, two adjacent alcohol O atoms bond to the π* orbital of the C=O group using the non-bonding electron pair (n) to form two H-O···C=O interactions, which are n (OH) →π* (CO) interactions ( Fig. 4d ). The HOMO (S 0 ) primarily consists of the non-bonding orbital of the C=O group (n (CO) , Fig. 4e ); therefore, the emission peaks located at 418 nm should be described as a n (OH) →π* (CO) stabilized S 1 →S 0 relaxation. The results from the calculations indicate that the H-O···C=O interaction has a significant role in stabilizing the excited state via an n (OH) →π* (CO) interaction, which results in a low-lying LUMO state and a red-shifted fluorescence. The results are consistent with those reported by Raines and co-workers [30] , in which theoretical calculations and high-resolution structures of green fluorescent proteins revealed the existence of a n→π* interaction between the chromophore of fluorescent proteins and a main-chain oxygen, and this interaction could contribute to the photophysical properties of the chromophore. Based on the above-mentioned results, the EDF behaviour can be explained by the electronically excited state manifold of the carbonyl groups due to the oscillating HO···C=O interactions caused by the collective proton motion system. Based on the results mentioned above, the n -EDFONPs are formed through radical-catalysed 3,2-acyl migration and stabilized by the hydrogen-bonded monoacylglycerol clusters with a collective proton motion and HO···C=O (n→π*) interactions. We suggest that the n -EDFONPs system could be considered as a model system of 2,2′-LBPA-rich organelles and could provide some biological implications in their formation and stabilization mechanisms, and biofunctions in late endosomes and lysosomes. The concept of 2-monoacylglycerol-induced EDFONP can be generalized to polymer systems. Replacing the reactant of 3,4,5-tris( n -alkyloxy) benzoic acid with the poly(ethylene glycol) bis(carboxymethyl) ether ( M n =600) resulted in an alternating copolymer, which is abbreviated as EDF-Polymer ( Fig. 5a and Supplementary Fig. S20a ). The molecular weight of the EDF-Polymer was estimated by gel-permeation chromatography and the number-average-molecular weight ( M n ) of the EDF-Polymer was ~12,000 Da. Emission spectrum of EDF-Polymer in CHCl 3 exhibits an EDF behaviour, which is similar to that of the n -EDFONPs ( Fig. 5b ), and the quantum yield is determined to be 6.1% with coumarin 1 as a reference. The HRTEM image reveals a aggregated nanoparticle with an approximately 5–8 nm diameter ( Fig. 5c ). We think that the nanoparticle of EDF-Polymer is constructed through a self-assembly process with bisphenol-A aggregates and poly(ethylene glycol) moieties serving as core and shell compartments, respectively ( Fig. 5d ). Future work will focus on the investigation of EDFONP as a biomimetic model of mono- or diacylglycerol-containing lipids and the potential applications of EDFONP and EDF-Polymer, especially for the fabrication of metal-free, low-cost organic/polymeric biosensing, bioimaging and optoelectronics materials. 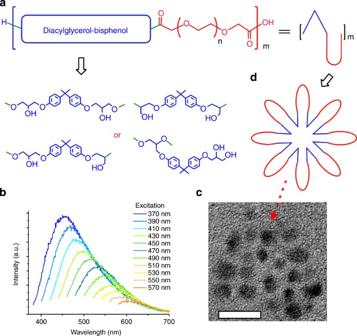Figure 5: Excitation-dependent fluorescent polymer. (a) Chemical structure of the EDF-Polymer. (b) Emission spectrum of the EDF-Polymer with a visible EDF phenomena. (c) HRTEM image shows an aggregated nanoparticles with a scale bar of 10 nm. (d) A cartoon model of nanoparticle with bisphenol-A aggregates and poly(ethylene glycol) moieties serving as core and shell compartments, respectively. Figure 5: Excitation-dependent fluorescent polymer. ( a ) Chemical structure of the EDF-Polymer. ( b ) Emission spectrum of the EDF-Polymer with a visible EDF phenomena. ( c ) HRTEM image shows an aggregated nanoparticles with a scale bar of 10 nm. ( d ) A cartoon model of nanoparticle with bisphenol-A aggregates and poly(ethylene glycol) moieties serving as core and shell compartments, respectively. Full size image Preparation of n -EDFONPs n -EDFONPs are prepared by two sequential reactions. The first reaction is a ring-opening reaction and the second reaction is a radical-catalysed 3,2-acyl migration reaction. General method for the synthesis of 12 -No-EDF via ring-opening reaction The preparation of 12 -No-EDF has been selected as a representative example, because the same procedure was systematically used for all the members of the series. A solution of bisphenol-A diglycidyl ether (0.68 g, 2.00 mmol), 3,4,5-tris(dodecyloxy)benzoic acid (2.80 g, 4.15 mmol) and tetra- n -butylammoium bromide (0.32 g, 1.00 mmol) in mix-solvent of acetonitrile (40 ml) and xylene (20 ml) was reflux at 85 °C for 24 h. The solvent was removed under reduced pressure. The crude product was recrystallized twice from ethanol, and a white solid is obtained (2.30 g, 68%) which is composed of 2,2′- 12 -BTBA and the 3,3′- 12 -BTBA positional isomers. 1 H NMR (600 MHz, CDCl 3 ): δ 7.26 (s, 4H), 7.14 (d, 4H, J =7.8 Hz), 6.83 (d, 4H, J =7.8 Hz), 5.41 (m, 0.34H, 2,2′- 12 -BTBA), 4.51 (m, 3.32H, 3,3′- 12 -BTBA), 4.34 (m, 1.66 H, 3,3′- 12 -BTBA), 4.26 (m, 0.68H, 2,2′- 12 -BTBA), 4.08 (m, 3.32H, 3,3′- 12 -BTBA), 4.02 (m, 12.68H,), 2.75 (b, 2H), 1.78 (m, 12H), 1.63 (s, 6H), 1.47 (m, 12H), 1.34 (m, 96H), 0.88 (t, 18H, J =6.6 Hz); 13 C NMR (150 MHz, CDCl3): δ 166.8, 156.2, 152.9, 143.8, 142.8, 127.6, 124.1, 114.0, 108.4, 77.1, 73.5, 69.3, 68.9 (3,3′- 12 -BTBA), 68.8(3,3′- 12 -BTBA), 66.4 (2,2′- 12 -BTBA), 66.1(3,3′- 12 -BTBA), 62.3 (2,2′- 12 -BTBA), 41.8, 31.9-22.7, 14.1; analysis (calcd., found for C 107 H 180 O 14 ): C (76.02, 76.01), H (10.73, 10.79). 14 -No-EDF, analysis (calcd., found for C 119 H 204 O 14 ): C (76.89, 76.87), H (11.06, 11.03). 16 -No-EDF, analysis (calcd., found for C 131 H 228 O 14 ): C (77.61, 77.23), H (11.34, 11.28). 18 -No-EDF, analysis (calcd., found for C 143 H 252 O 14 ): C (78.23, 77.94), H (11.57, 11.58). The DEPT-135, HSQC and HMBC spectra are shown in Supplementary Figs S1–S3 . General method for the synthesis of 12 -EDFONPs via radical-catalysed 3,2-acyl migration reaction The preparation of 12 -EDFONP has been selected as a representative example because the same procedure was systematically used for all the members of the series. 12 -No-EDF (0.7402, g, 0.44 mmol) and ammonium persulphate (0.013 g, 0.057 mmol) were heated and stirred under N 2 at 150 °C for 38 h. The crude product was then disolved in CH 2 Cl 2 and filtered. The filtrate was dried under vacuum to give a brown product with a yield of 97% (0.72 g, 0.43 mmol), which is composed of 2,2′- 12 -BTBA, 2,3- 12 -BTBA, 3,3′- 12 -BTBA and 2,3- 12 -diacylglycerol-bisphenol-glycerol isomers, and no any non-acyl-migrated side product is found. 1 H NMR (600 MHz, CDCl 3 ): δ 7.27 (b, 4H), 7.11 (b, 4H), 6.88 (b, 4H), 5.73 (s, 0.04H), 5.52 (s, 1.2H), 5.42 (s, 0.02H), 4.78 (m, 0.04H), 4.66 (m, 0.04H), 4.52 (b, 1.4H), 4.36 (b, 0.3H), 4.11 (b, 18.96H), 1.76 (m, 12H), 1.60 (s, 6H), 1.46 (m, 12H), 1.27 (m, 96H), 0.87 (t, 18H, J =6.6 Hz); 13 C NMR (150 MHz, CDCl3): δ 170.9, 160.1, 143.8, 143.1, 127.8, 124.2, 114.4, 108.2, 77.1, 73.5, 71.8, 70.2, 69.2, 68.9, 68.7, 68.9, 67.9, 66.3, 64.4, 63.3, 62.3, 41.8, 31.9, 31.1, 30.4, 29.6, 26.1, 22.7, 14.1; analysis (calcd., found for C 107 H 180 O 14 ): C (76.02, 76.74), H (10.73, 10.74). 14 -EDFONP, analysis (calcd., found for C 119 H 204 O 14 ): C (76.89, 77.34), H (11.06, 11.07). 16 -EDFONP, analysis (calcd., found for C 131 H 228 O 14 ): C (77.61, 77.91), H (11.34, 11.38). 18 -EDFONP, analysis (calcd., found for C 143 H 252 O 14 ): C (78.23, 78.62), H (11.57, 11.57). The 1 H, 13 C DEPT-135, 1 H– 13 C HSQC and HMBC spectra are shown in Supplementary Figs S4–S12 . Synthesis and compound characterization Synthesis and characterization of 17 -EDFONP, 16 - BGE-EDFONP- and EDF-Polymer are described in Supplementary Methods . How to cite this article: Lee, K-M. et al. Excitation-dependent visible fluorescence in decameric nanoparticles with monoacylglycerol cluster chromophores. Nat. Commun. 4:1544 doi: 10.1038/ncomms2563 (2013).